Structural basis of allosteric interactions among Ca2+-binding sites in a K+channel RCK domain Ligand binding sites within proteins can interact by allosteric mechanisms to modulate binding affinities and control protein function. Here we present crystal structures of the regulator of K + conductance (RCK) domain from a K + channel, MthK, which reveal the structural basis of allosteric coupling between two Ca 2+ regulatory sites within the domain. Comparison of RCK domain crystal structures in a range of conformations and with different numbers of regulatory Ca 2+ ions bound, combined with complementary electrophysiological analysis of channel gating, suggests chemical interactions that are important for modulation of ligand binding and subsequent channel opening. Regulator of K + conductance (RCK) domains control the activity of a variety of K + channels and transporters, including the prokaryotic TrkA/H K + transport complex and the eukaryotic large-conductance calcium-activated (BK) channel, through binding of cytoplasmic ligands such as ATP, H + and Ca 2+ (refs 1 , 2 , 3 , 4 , 5 , 6 , 7 , 8 ). Thus, RCK domains transduce ligand binding to gate transmembrane K + flux in response to signalling events and cellular metabolism, in organisms ranging from bacteria to humans. In addition, binding of one ligand to an RCK domain can allosterically modulate binding of a second ligand, resulting in tuning of channel or transporter activity in response to cellular stimuli [9] , [10] , [11] . These allosteric interactions are key in generating a wide dynamic range for ligand activation of channels and transporters, in addition to linking multiple stimulus modalities to gate ion flux. Although allosteric interactions in the RCK domains have been described in functional terms, the structural bases for such interactions are yet unclear [10] , [12] , [13] . Using electrophysiology and X-ray crystallography, we address the structural basis of allosteric interaction among Ca 2+ -binding sites in the MthK Ca 2+ -gated K + channel. MthK is a prototypical K + channel, whose crystal structure has provided insight towards mechanisms of channel gating by RCK domains [4] , [9] , [10] , [14] , [15] , [16] , [17] , [18] . In MthK, binding of cytoplasmic Ca 2+ to a tethered octameric ring of RCK domains (the ‘gating ring’) leads to a series of conformational changes that facilitates channel opening and K + conduction [4] , [10] , [19] , [20] , [21] . Here, by solving structures of mutant and wild-type (WT) RCK domains, we find that distinct Ca 2+ activation sites near the amino and carboxy termini of the RCK domain (termed C1 and C3, respectively) are allosterically coupled to one another, to affect tuning of Ca 2+ affinity and Ca 2+ -dependent channel activation. These results define a structural mechanism of allosteric modulation in a ligand-gated K + channel, and provide a framework for understanding similar mechanisms in related RCK-containing channels and transporters. The E212Q mutation paradoxically enhances Ca 2+ sensitivity MthK contains three Ca 2+ -binding sites per RCK domain that facilitate channel activation (termed C1, C2 and C3; Fig. 1 ) [16] . Consistent with the activating role of Ca 2+ , we observe that charge neutralization of the Ca 2+ -coordinating side chains D184 and E210 at the Ca 2+ -binding site C1 leads to MthK channels with decreased Ca 2+ sensitivity; the [Ca 2+ ] yielding half-maximal channel open probability (EC 50 ) was 2.2±0.1 mM for WT ( n =5), 6.3±0.4 mM for D184N ( n =5) and 4.0±0.3 mM for E210Q ( n =6), all at pH 7.7 (throughout, EC 50 values reported for each mutant are the means of EC 50 values determined from individual patches±s.e.m.). However, neutralization of the Ca 2+ -coordinating side chain E212 at the same binding site yields channels with increased Ca 2+ sensitivity (EC 50 =1.3±0.1 mM Ca 2+ for E212Q, n =8, pH 7.7; Fig. 1f ). Ca 2+ activation of MthK is known to be sensitive to pH, and these mutant effects persisted at pH 6.5 (EC 50 =16±1.6 mM Ca 2+ for WT, n =6; 30±2.0 mM Ca 2+ for D184N, n =7; and 9.9±0.3 mM Ca 2+ for E212Q, n =5; Fig. 1g ); although increasing [H + ] leads to an overall shift in EC 50 toward higher [Ca 2+ ], the E212Q mutant consistently requires less Ca 2+ for activation than MthK WT. 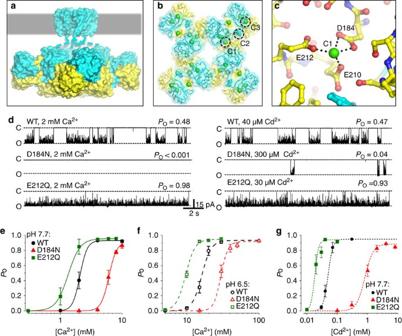Figure 1: Functional effects of mutations at Ca2+-binding site C1. (a) Structure of the MthK channel shown as surface rendering (PDB accession number3RBZ). The pore (in the plasma membrane, represented by grey shading) and its contiguous RCK domains (at the cytoplasmic side) are coloured cyan; dashed cyan lines represent the unresolved pore–RCK linker residues. Associated RCK domains (which complete the gating ring complex) are coloured yellow. (b) Cα trace of the gating ring superimposed within its surface rendering as viewed from above the membrane; the pore has been removed for clarity. RCK domains are coloured as ina; Ca2+ions are shown as green spheres. Locations of representative C1, C2 and C3 Ca2+ions are indicated by circles. (c) Magnified view of the C1 Ca2+-binding site; dashed lines indicate coordination by oxygens from carboxylate side chains of D184, E210 and E212. (d) Representative single-channel current traces from WT and C1 mutant MthK channels, at indicated [Ca2+]i(left) or [Cd2+]i(right). D184N channels show reduced Ca2+and Cd2+sensitivity, but E212Q channels show enhanced sensitivity. These and subsequent current traces were recorded in symmetrical 200 mM KCl, Vm=−100 mV. (e) Activation of WT, D184N and E212Q channels by Ca2+at pH 7.7 (WT,n=5; D184N,n=5; and E212Q,n=8). (f) Activation of WT, D184N and E212Q channels by Ca2+at pH 6.5 (WT,n=6; D184N,n=7; and E212Q,n=5). (g) Activation of WT, D184N and E212Q channels by Cd2+at pH 7.7 (WT,n=8; D184N,n=6; and E212Q,n=5). Data points indicate mean Po±s.e.m. at the indicated ligand concentration. Figure 1: Functional effects of mutations at Ca 2+ -binding site C1. ( a ) Structure of the MthK channel shown as surface rendering (PDB accession number 3RBZ ). The pore (in the plasma membrane, represented by grey shading) and its contiguous RCK domains (at the cytoplasmic side) are coloured cyan; dashed cyan lines represent the unresolved pore–RCK linker residues. Associated RCK domains (which complete the gating ring complex) are coloured yellow. ( b ) Cα trace of the gating ring superimposed within its surface rendering as viewed from above the membrane; the pore has been removed for clarity. RCK domains are coloured as in a ; Ca 2+ ions are shown as green spheres. Locations of representative C1, C2 and C3 Ca 2+ ions are indicated by circles. ( c ) Magnified view of the C1 Ca 2+ -binding site; dashed lines indicate coordination by oxygens from carboxylate side chains of D184, E210 and E212. ( d ) Representative single-channel current traces from WT and C1 mutant MthK channels, at indicated [Ca 2+ ] i (left) or [Cd 2+ ] i (right). D184N channels show reduced Ca 2+ and Cd 2+ sensitivity, but E212Q channels show enhanced sensitivity. These and subsequent current traces were recorded in symmetrical 200 mM KCl, Vm=−100 mV. ( e ) Activation of WT, D184N and E212Q channels by Ca 2+ at pH 7.7 (WT, n =5; D184N, n =5; and E212Q, n =8). ( f ) Activation of WT, D184N and E212Q channels by Ca 2+ at pH 6.5 (WT, n =6; D184N, n =7; and E212Q, n =5). ( g ) Activation of WT, D184N and E212Q channels by Cd 2+ at pH 7.7 (WT, n =8; D184N, n =6; and E212Q, n =5). Data points indicate mean Po±s.e.m. at the indicated ligand concentration. Full size image Aside from Ca 2+ , MthK channels can also be activated by Cd 2+ with EC 50 in the micromolar range, through binding of Cd 2+ ions at the C1 and C3 activation sites [21] , [22] , [23] . Figure 1 illustrates that the MthK WT channel is activated by Cd 2+ with an EC 50 of 49.1±5.0 μM ( n =8). The functional effects of the D184N and E212Q mutations on Cd 2+ activation, indicated by the shift in EC 50 , were even stronger than their effects on Ca 2+ activation. D184N channels were activated with an EC 50 of 880±80 μM Cd 2+ ( n =6, an 18-fold increase in EC 50 compared with that in WT), whereas E212Q channels were activated with an EC 50 of 16.3±2.9 μM Cd 2+ ( n =5; a 3-fold decrease in EC 50 compared with that in WT). Charge-neutralizing mutation is a commonly used approach towards identifying Ca 2+ -coordinating side chains in proteins [24] , [25] , [26] , [27] . Thus, our initial goal in the present work was to learn the relation between these mutation effects and the Ca 2+ -activation mechanism in MthK, in part by solving crystal structures of binding-site mutants in the presence of Ca 2+ . Effects of Ca 2+ on RCK domain conformation To gain insight towards the structures of the Ca 2+ -binding sites in the MthK RCK domain, we crystallized the RCK domain in the presence of Ca 2+ , in a crystal form that diffracted X-rays to 2.5 Å, in space group P3 1 21 ( Fig. 2 ). The structure was solved by molecular replacement and refined to R work / R free of 0.178/0.226 ( Table 1 ). As strong electron density peaks were observed at each of the three Ca 2+ activation sites, termed C1, C2 and C3, we refer to this structure as WT-C1C2C3. The Ca 2+ -bound RCK domains in this structure form a dimer, with each peptide chain consisting of an N-lobe, a domain-swapping helix-turn-helix motif and a C-lobe ( Fig. 2a ). In this context, it can be seen that the C1 site is contained entirely within a single N-lobe ( Fig. 2b ), whereas the Ca 2+ ion of the C2 site forms an intersubunit bridge between the ‘turn’ of the helix-turn-helix motif and the C-lobe of adjacent subunits ( Fig. 2c ), and the Ca 2+ ion of the C3 site also forms an intersubunit bridge between C-lobes of adjacent subunits ( Fig. 2d ). 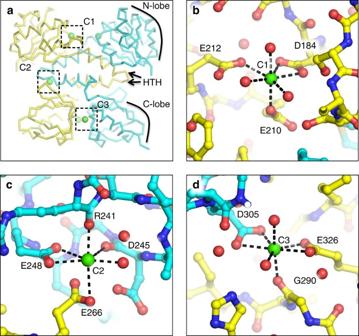Figure 2: Structural details of Ca2+activation sites at 2.5 Å. (a) Schematic representation of the RCK domain dimer. Component subunits are coloured cyan and yellow; Ca2+ions and water are represented by green and red spheres, respectively. Locations of the N-lobe, helix-turn-helix (HTH) and C-lobe are as indicated. Dashed boxes indicate locations of Ca2+sites. (b–d) Ball and stick representations of Ca2+sites C1 (b), C2 (c) and C3 (d). Ca2+coordination is illustrated by dashed lines. Figure 2: Structural details of Ca 2+ activation sites at 2.5 Å. ( a ) Schematic representation of the RCK domain dimer. Component subunits are coloured cyan and yellow; Ca 2+ ions and water are represented by green and red spheres, respectively. Locations of the N-lobe, helix-turn-helix (HTH) and C-lobe are as indicated. Dashed boxes indicate locations of Ca 2+ sites. ( b – d ) Ball and stick representations of Ca 2+ sites C1 ( b ), C2 ( c ) and C3 ( d ). Ca 2+ coordination is illustrated by dashed lines. Full size image Table 1 Data collection and refinement statistics. 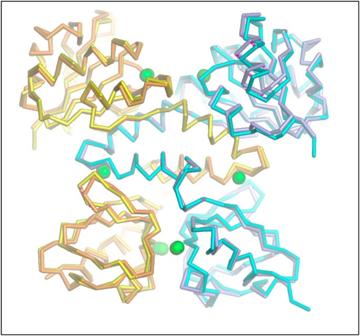Figure 3: Alignment of RCK dimers from WT-C1C2C3 and Ca2+-bound MthK channel. Overlayed Cα traces of WT-C1C2C3 (yellow/cyan) and RCK domains from Ca2+-bound MthK channel (PDB accession number3RBZ; orange/purple). The small overall root mean squared difference for these aligned structures (0.8 Å) suggests that they represent nearly identical conformations. Full size table It is worth noting that the overall conformation of the WT-C1C2C3 structure recapitulates the RCK domain conformation within the gating ring of the Ca 2+ -bound, open MthK channel, although the WT-C1C2C3 structure did not itself crystallize as a gating ring, and the WT-C1C2C3 crystals are comprises the RCK domain only, not tethered to the MthK pore ( Figure 3 ) [4] , [16] . The similarity between the WT-C1C2C3 structure and the RCK domains from the fully liganded open channel is thus consistent with the idea that the domain conformation depends primarily on Ca 2+ occupancy at the activation sites, and is not strictly dependent on tethering to the MthK pore or formation of the gating ring complex. Figure 3: Alignment of RCK dimers from WT-C1C2C3 and Ca 2+ -bound MthK channel. Overlayed Cα traces of WT-C1C2C3 (yellow/cyan) and RCK domains from Ca 2+ -bound MthK channel (PDB accession number 3RBZ ; orange/purple). The small overall root mean squared difference for these aligned structures (0.8 Å) suggests that they represent nearly identical conformations. Full size image The WT-C1C2C3 structure defines previously unresolved details of ion coordination within the domain’s Ca 2+ activation sites. For example, the Ca 2+ ion at each site was surrounded by protein oxygens and ordered solvent molecules, exhibiting canonical bipyramidal coordination geometries ( Fig. 2 ) [16] , [28] , [29] , [30] . Notably, the C2 Ca 2+ ion is seen to be coordinated at the centre of a ring formed by side-chain oxygens from residue E248, the carbonyl oxygen from D245 and a water of hydration, with the capstones of each pyramid formed by a side-chain oxygen from E266 and the carbonyl oxygen from R241. Similarly, the C3 Ca 2+ ion is coordinated at the centre of a ring formed by side-chain oxygens from residues D305 and E326, and one water of hydration, with a carbonyl oxygen from G290 and a second water of hydration forming the capstones of each pyramid. Finally, the C1 Ca 2+ ion is at the centre of a ring formed by two oxygen atoms from the D184 side chain, two water molecules and one oxygen atom from the E212 side chain [28] . As both D184 and E212 directly coordinate the Ca 2+ ion at C1 in the context of the fully liganded RCK domain, one might predict that neutralization of D184 or E212 by mutation to N or Q, respectively, would weaken the electrostatic interaction with Ca 2+ in both cases, and thus decrease Ca 2+ -dependent channel activation. Although the D184N mutation decreases Ca 2+ activation, the E212Q mutation unexpectedly increases Ca 2+ activation ( Fig. 1 ). We next addressed the structural basis of these functional effects. Crystal structures of gating mutants To determine whether mutations at the C1 site affect only Ca 2+ binding at C1 or, alternatively, have allosteric effects at other Ca 2+ -binding sites, we sought to compare the structures of WT and mutant RCK domains, crystallized under the same conditions as one another, to minimize the contribution of differences in pH or ionic strength to structural changes that might be observed. To find conditions that would allow such direct comparison of mutant and WT domain structures, we started with the crystallization buffer that yielded the WT-C1C2C3 structure and examined crystals formed with lower [Ca 2+ ] to yield WT crystals in which not all Ca 2+ sites were occupied. When [Ca 2+ ] was lowered within the range of 20–300 mM CaCl 2 in this crystallization buffer, WT RCK domains crystallized in space group P2 1 and contained a Ca 2+ ion bound only at the C1 site. The C3 sites in this structure are in conformations that are different from the C3-bound structure ( Fig. 4a,b compared with Fig. 2b,d ). Although one cannot determine binding constants from these data, the observation that lowering [Ca 2+ ] leads to dissociation of Ca 2+ from C3 but not C1 is consistent with C1 being the higher-affinity site under these conditions. This structure, termed WT-C1 (formed in 200 mM Ca 2+ ), was refined to 1.85 Å resolution with R work / R free of 0.211/0.253 ( Table 1 ). The crystallization conditions for WT-C1 were then used as a template for crystallization of the D184N and E212Q mutant RCK domains. 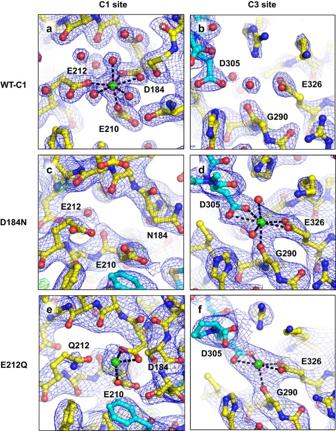Figure 4: Effects of Ca2+on conformation of WT and mutant RCK domains. (a,b) Structures of the C1 and C3 sites from the WT RCK domain crystallized with 0.2 M Ca2+, overlayed with 2Fo–Fc map contoured at 1.2σ (blue mesh) and 5σ (purple mesh). (c,d) Structures of the same regions from the D184N mutant RCK domain, overlayed with 2Fo–Fc map contoured at 1.2σ (blue mesh) and Fo–Fc map contoured at 4σ (positive peaks shown as green mesh), indicating the absence of significant unmodelled electron density at the C1 site. (e) Structure of the C1 site from the E212Q mutant RCK domain crystallized under the same conditions as WT-C1, overlayed with 2Fo–Fc map contoured at 1.5σ (blue mesh). (f) Structure of the C3 site from the E212Q mutant RCK domain, overlayed with 2Fo–Fc map contoured at 1.5σ (blue mesh) and 5σ (purple mesh). Maps were calculated using data to 1.85 Å (a,b), 2.4 Å (c,d) and 3.0 Å resolution (e,f). Figure 4: Effects of Ca 2+ on conformation of WT and mutant RCK domains. ( a , b ) Structures of the C1 and C3 sites from the WT RCK domain crystallized with 0.2 M Ca 2+ , overlayed with 2Fo–Fc map contoured at 1.2σ (blue mesh) and 5σ (purple mesh). ( c , d ) Structures of the same regions from the D184N mutant RCK domain, overlayed with 2Fo–Fc map contoured at 1.2σ (blue mesh) and Fo–Fc map contoured at 4σ (positive peaks shown as green mesh), indicating the absence of significant unmodelled electron density at the C1 site. ( e ) Structure of the C1 site from the E212Q mutant RCK domain crystallized under the same conditions as WT-C1, overlayed with 2Fo–Fc map contoured at 1.5σ (blue mesh). ( f ) Structure of the C3 site from the E212Q mutant RCK domain, overlayed with 2Fo–Fc map contoured at 1.5σ (blue mesh) and 5σ (purple mesh). Maps were calculated using data to 1.85 Å ( a , b ), 2.4 Å ( c , d ) and 3.0 Å resolution ( e , f ). Full size image The D184N RCK domain crystallized in space group P6 5 22 and the structure was refined to 2.4 Å resolution with R work / R free of 0.197/0.247 ( Table 1 ). In this structure, no electron density that could be modelled as a Ca 2+ ion was detectable at C1 ( Fig. 4c ). However, interestingly, density corresponding to Ca 2+ ions was clearly observed at C3; the resolution of these data was sufficient to resolve ordered solvent surrounding the Ca 2+ ions at C3, recapitulating the coordination geometry observed in the WT-C1C2C3 structure ( Fig. 4d , compared with Fig. 2d ). As the [Ca 2+ ] in the D184N crystallization buffer was the same as that in the WT-C1 buffer, these results suggest that the D184N mutation has altered the relative affinities of the C1 and C3 sites for Ca 2+ . This observation further suggests that these two Ca 2+ sites are allosterically coupled to one another, that is, the D184N mutation, which directly alters Ca 2+ binding at the C1 site, also effects Ca 2+ binding at the physically distinct C3 site. To gain further insight towards the allosteric relation between C1 and C3, we crystallized the E212Q RCK domain. This mutant also crystallized in space group P6 5 22 and the structure was refined to 3.0 Å resolution with R work / R free of 0.217/0.263. In contrast to D184N, the E212Q mutant did contain electron density at the C1 and C3 site, modelled as Ca 2+ ( Figs 4e,f and 5 ). Interestingly, however, Ca 2+ coordination at the C1 site of the E212Q mutant is different from the configuration of the C1 site in the WT-C1 or WT-C1C2C3 structures. At the WT C1 site, the E212 side chain appears to directly coordinate Ca 2+ , with a mean Ca 2+ –Oε distance of ~2.5 Å ( Figs 1c and 4a ) [16] , [28] . In contrast, the nearest Oε/Nε atoms from Q212 are further from Ca 2+ than the canonical coordination distance (mean distance=3.3 Å; Fig. 4e ), suggesting that Q212 does not participate in direct coordination of the C1 Ca 2+ ion. The distance between Ca 2+ and the other key oxygen ligands, from the D184 and E210 side chains, are similar to those observed in the WT-C1 or WT-C1C2C3 structures ( Figs 2b and 4a ; mean distances for E212Q structure were 2.6 Å for D184/Oδ and 2.5 Å for E210/Oε). Thus, the position of the Q212 side chain in the E212Q mutant may be less constrained by Ca 2+ coordination than the E212 side chain in the WT RCK domain. As the E212 side chain would similarly be unconstrained by Ca 2+ in the D184N mutant, Ca 2+ coordination by the E212 side chain may be important in allosteric coupling between the C1 and C3 Ca 2+ -binding sites. 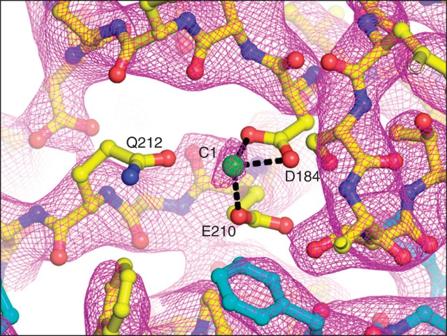Figure 5: Omit map of the C1 site from the E212Q mutant RCK domain is consistent with a bound Ca2+ion at the site. To further validate modelling of Ca2+ions at the C1 site in the E212Q structure, we calculated omit maps to minimize bias arising from model-derived phase information. The complete structure of the E212Q C1 site is shown in ball and stick representations, with Ca2+ion as green spheres. The omit map (purple mesh, contoured at 1.5σ) was calculated by omitting Ca2+ions and surrounding side chains (D184, E210 and Q212) from this structure, then performing simulated annealing refinement to eliminate the contribution of the omitted atoms in the calculation of phase information. The position of the electron density peak in the omit map that coincides with the position of the Ca2+ion in the complete structure is thus consistent with the presence of Ca2+at the site. Figure 5: Omit map of the C1 site from the E212Q mutant RCK domain is consistent with a bound Ca 2+ ion at the site. To further validate modelling of Ca 2+ ions at the C1 site in the E212Q structure, we calculated omit maps to minimize bias arising from model-derived phase information. The complete structure of the E212Q C1 site is shown in ball and stick representations, with Ca 2+ ion as green spheres. The omit map (purple mesh, contoured at 1.5σ) was calculated by omitting Ca 2+ ions and surrounding side chains (D184, E210 and Q212) from this structure, then performing simulated annealing refinement to eliminate the contribution of the omitted atoms in the calculation of phase information. The position of the electron density peak in the omit map that coincides with the position of the Ca 2+ ion in the complete structure is thus consistent with the presence of Ca 2+ at the site. Full size image The effect of mutation on Ca 2+ -binding at sites C1 and C3 observed in the D184N and E212Q crystal structures suggest a mechanism underlying the functional effects of these mutations on Ca 2+ -dependent gating of MthK. Ca 2+ binding at C1, which appears to be the higher-affinity site in the WT RCK domain, makes Ca 2+ binding at C3 relatively unfavourable ( Fig. 4a,b ). The D184N mutation, which abrogates Ca 2+ binding at C1, makes Ca 2+ binding at C3 more favourable than it is in WT under the same conditions; however, the apparent loss of Ca 2+ binding at C1 results in an overall decreased Ca 2+ sensitivity of the D184N mutant channel ( Figs 1d–g and 4c ). As the E212Q mutation also makes Ca 2+ binding at C3 more favourable than it is in WT, but does not eliminate Ca 2+ binding at C1, Ca 2+ activation of E212Q channels is enhanced over that of the WT ( Figs 1d–g and 3e,f ). Structural basis of allosteric coupling We reasoned that if C1 and C3 are allosterically coupled to one another, then they must be linked through a series of chemical bonds such that Ca 2+ binding at C1 raises the energy barrier for Ca 2+ binding at C3. Thus, we hypothesized that interactions (for example, salt bridges or hydrogen bonds) in the RCK domain that are correlated with occupancy or vacancy of C3 may determine part of the physical link between these sites and may underlie their allosteric modulation. To test this hypothesis, we systematically compared the structures of WT-C1, WT-C1C2C3, D184N and E212Q with the goal of identifying specific chemical bonds that are correlated with the presence or absence of Ca 2+ at C3. Among the potential polar and electrostatic interactions present in the MthK RCK domain, the side chains of E133 and E259 in WT-C1 had Oε–Oε distances of 2.8 Å, consistent with a carboxyl–carboxylate hydrogen bond (that is, <3.2 Å; Fig. 6 ). In contrast, these Oε–Oε distances were much greater in the WT-C1C2C3, D184N and E212Q structures (WT-C1C2C3, 6.2 Å; D184N, 7.3 Å; and E212Q, 8.3 Å; Figs 6 and 7 ). To test further whether the hydrogen bonding observed with WT-C1 was present or absent in previous MthK structures, we examined structures of the RCK domain crystallized with 0 and 20 mM Ca 2+ (PDB accession numbers 2AEJ and 2AEF , solved to 2.1 and 1.7 Å resolution, respectively) [28] . In these structures, minimum Oε–Oε distances for E133–E259 were 3.1 Å and 2.8 Å for 0 and 20 mM Ca 2+ , respectively ( Fig. 7 ). 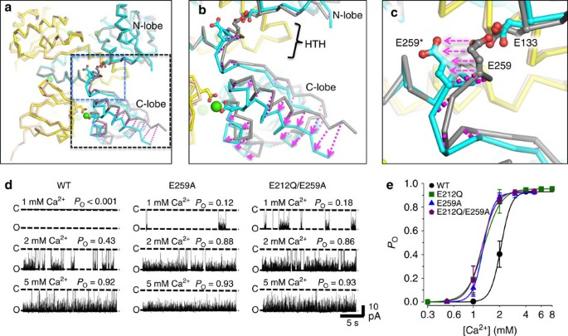Figure 6: E259 forms a pivot point to gate Ca2+-dependent RCK domain activation. (a) Aligned Cα traces of WT-C1 (dark yellow/grey) and WT-C1C2C3 (light yellow/cyan) illustrating apparent movement of the C-lobe (inside black dashed box) and E259 side chain (inside blue dashed box) relative to other regions. (b) Expanded view of the large boxed region ina, with magenta dashed arrows indicating the direction of apparent Ca2+-dependent movement. (c) Expanded view of the smaller boxed region ina, with magenta dashed arrows indicating the direction of the apparent movement of the E259 side chain, relative to E133; E259* indicates the E259 side chain from WT-C1C2C3, with Ca2+bound at C3. (d) Representative single-channel current traces of MthK WT, E259A and E212Q/E259A mutant channels over a range of [Ca2+]. Channels containing the E259A mutation alone or in combination with E212Q show enhanced Ca2+sensitivity compared with WT. (e) Po versus [Ca2+] for WT and mutant channels. Data points indicate mean Po±s.e.m. Activation curves for E212Q (n=8), E259A (n=5) and E212Q/E259A channels (n=5) are each shifted towards lower [Ca2+] relative to WT, consistent with decreased inhibitory coupling. Figure 6: E259 forms a pivot point to gate Ca 2+ -dependent RCK domain activation. ( a ) Aligned Cα traces of WT-C1 (dark yellow/grey) and WT-C1C2C3 (light yellow/cyan) illustrating apparent movement of the C-lobe (inside black dashed box) and E259 side chain (inside blue dashed box) relative to other regions. ( b ) Expanded view of the large boxed region in a , with magenta dashed arrows indicating the direction of apparent Ca 2+ -dependent movement. ( c ) Expanded view of the smaller boxed region in a , with magenta dashed arrows indicating the direction of the apparent movement of the E259 side chain, relative to E133; E259* indicates the E259 side chain from WT-C1C2C3, with Ca 2+ bound at C3. ( d ) Representative single-channel current traces of MthK WT, E259A and E212Q/E259A mutant channels over a range of [Ca 2+ ]. Channels containing the E259A mutation alone or in combination with E212Q show enhanced Ca 2+ sensitivity compared with WT. ( e ) Po versus [Ca 2+ ] for WT and mutant channels. Data points indicate mean Po±s.e.m. Activation curves for E212Q ( n =8), E259A ( n =5) and E212Q/E259A channels ( n =5) are each shifted towards lower [Ca 2+ ] relative to WT, consistent with decreased inhibitory coupling. 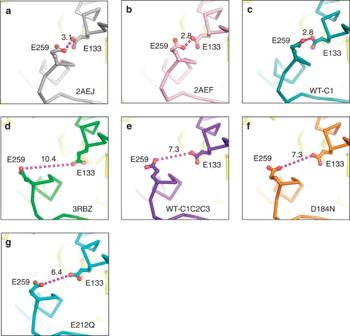Figure 7: Distances between E259 and E133 side chains in MthK crystal structures. (a–g) Cα traces of the indicated structures with E259 and E133 side chains shown as ball and stick representations. The minimal distances (in Å) between E259 and E133 Oε atoms are indicated by dashed magenta lines. The shortest distances among these, consistent with a hydrogen bond length (<3.2 Å), are associated with structures in which no Ca2+is bound at the C3 site (a–c). In contrast, longer distances are associated with structures of WT (d,e) or mutant RCK domains (f,g) in conditions where Ca2+ions are bound at the C3 site. Structures inaandb(PDB accession numbers2AEJand2AEF, respectively) are from ref.28; structure ind(PDB accession number3RBZ) is from ref.16. Full size image Figure 7: Distances between E259 and E133 side chains in MthK crystal structures. ( a – g ) Cα traces of the indicated structures with E259 and E133 side chains shown as ball and stick representations. The minimal distances (in Å) between E259 and E133 Oε atoms are indicated by dashed magenta lines. The shortest distances among these, consistent with a hydrogen bond length (<3.2 Å), are associated with structures in which no Ca 2+ is bound at the C3 site ( a – c ). In contrast, longer distances are associated with structures of WT ( d , e ) or mutant RCK domains ( f , g ) in conditions where Ca 2+ ions are bound at the C3 site. Structures in a and b (PDB accession numbers 2AEJ and 2AEF , respectively) are from ref. 28 ; structure in d (PDB accession number 3RBZ ) is from ref. 16 . Full size image The close proximity between the E133 and E259 side chains in the WT-C1 structure and the previous structures with 0 and 20 mM Ca 2+ predicts that these side chains are at least partially protonated; if these side chains were deprotonated, both would carry negative charges, and thus repel one another. Although the WT-C1C2C3, D184N and E212Q structures each show greater Oε–Oε distances for these side chains compared with WT-C1, it should be noted that all of these crystals were grown at the same pH. Thus, the differences in conformation are not likely to arise from differences in side-chain protonation. Together, these results suggest that the E133–E259 interaction is correlated with the absence of Ca 2+ occupancy at C3; however, it is not clear from these structural observations alone whether this interaction is related to channel gating. We next tested whether the E133–E259 interaction affects channel gating, by assaying the Ca 2+ -activation properties of the E259A mutant channels, designed to constitutively disrupt the carboxyl–carboxylate interaction. We observe that the E259A-gating phenotype was very similar to E212Q, with EC 50 values that were shifted towards lower [Ca 2+ ] compared with WT (mean EC 50 =1.4±0.1 mM Ca 2+ , n =5; Fig. 6d,e ). This electrophysiological result is consistent with the idea that the E259 side chain contributes to inhibitory coupling between C1 and C3. If E212 and E259 each contribute to allosteric coupling between C1 and C3, then one might predict that the combined effects of the E212Q and E259A mutations on Ca 2+ activation of the channel would be energetically non-additive [31] . To test this, we assayed Ca 2+ activation of the E212Q/E259A double mutant and found that the EC 50 of this double mutant (1.4±0.2 mM Ca 2+ , n =5) was not significantly different from either the E212Q or E259A single mutants ( Fig. 6e ). Although we cannot yet rule out that other modulatory interactions exist, the observation that the E212Q/E259A double mutant is effectively indistinguishable from the single mutants suggests that either disruption of the direct E212-Ca 2+ bond or the E259–E133 hydrogen bond is sufficient to disrupt allosteric communication between these sites. Here we have used electrophysiological and crystallographic analysis of MthK to dissect potential mechanisms underlying activation and modulation of RCK domains. We observe principally that two physically distinct Ca 2+ -binding sites on the RCK domain are structurally and energetically coupled to one another, and we further define a key interaction that mediates this allosteric coupling to tune Ca 2+ sensitivity of the channel. A working hypothesis for the allosteric coupling mechanism is illustrated in Fig. 8 . In this scheme, with Ca 2+ -binding sites empty ( Fig. 8a ), the RCK domains may exist in a range of conformations, as observed in structures of the unliganded MthK gating ring [17] , [21] . Ca 2+ binding at the C1 sites (in the N-lobes) would then lead to stabilization of a partially activated conformation [16] , [21] ( Fig. 8b ). Structures of WT and mutant RCK domains that display differences in Ca 2+ occupancy at the C1 and C3 sites (and different overall conformations) further suggest that movements of the N-lobe and C-lobe are coupled to one another, attributable in part to an apparent carboxyl–carboxylate hydrogen bond between E133 and E259 ( Figs 6 and 7 ). With the E133–E259 interaction intact, the Ca 2+ -bound conformation of the N-lobe is incompatible with Ca 2+ binding to the C3 sites ( Figs 6 and 7 ). Thus, it appears that Ca 2+ binding at C3 requires either disruption of the E133–E259 interaction ( Fig. 8c ), as with the E259A mutation, or disruption of Ca 2+ coordination at C1, as with the D184N and E212Q mutations ( Figs 4 and 5 ). Ca 2+ occupancy at both the C1 and C3 sites is required for complete activation of the RCK domain and maximal stabilization of channel opening. 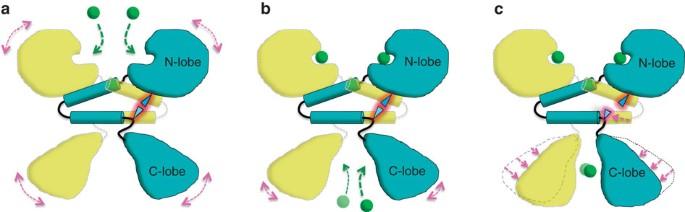Figure 8: Working hypothesis for allosteric interaction in the RCK domain. (a) With Ca2+-binding sites empty, the RCK domains may exist in a range of conformations (represented by dashed magenta arrows). Movements of the N-lobe and C-lobe are coupled to one another, due in part to the E133–E259 carboxyl–carboxylate bond (blue triangles, highlighted in red). Ca2+ions (green spheres) initially bind to the C1 sites in the N-lobe of each domain. (b) With Ca2+bound at the C1 sites, a partially activated conformation is stabilized, but Ca2+binding to the C3 sites is blunted, due in part to the E133–E259 interaction. (c) Increasing [Ca2+] further leads to Ca2+binding to the C3 sites, which bridge the C-lobes of adjacent RCK domains. The conformational change associated with C3 binding involves movements of E259 and the C-lobe (represented by magenta highlighting and dashed arrows, respectively). Figure 8: Working hypothesis for allosteric interaction in the RCK domain. ( a ) With Ca 2+ -binding sites empty, the RCK domains may exist in a range of conformations (represented by dashed magenta arrows). Movements of the N-lobe and C-lobe are coupled to one another, due in part to the E133–E259 carboxyl–carboxylate bond (blue triangles, highlighted in red). Ca 2+ ions (green spheres) initially bind to the C1 sites in the N-lobe of each domain. ( b ) With Ca 2+ bound at the C1 sites, a partially activated conformation is stabilized, but Ca 2+ binding to the C3 sites is blunted, due in part to the E133–E259 interaction. ( c ) Increasing [Ca 2+ ] further leads to Ca 2+ binding to the C3 sites, which bridge the C-lobes of adjacent RCK domains. The conformational change associated with C3 binding involves movements of E259 and the C-lobe (represented by magenta highlighting and dashed arrows, respectively). Full size image An inhibitory interaction between two Ca 2+ -binding sites in the same protein may represent a structural mechanism that underlies ‘tuning’ of the protein’s Ca 2+ sensitivity. In the case of MthK, crystallographic structures indicate that the C1 site, located within the N-lobe of each RCK domain, undergoes relatively subtle structural changes upon Ca 2+ binding and appears to bind Ca 2+ with higher relative affinity than the C3 site ( Fig. 4a,b ) [16] , [28] . Thus, in conditions where Ca 2+ binding at C1 inhibits binding at C3, a Ca 2+ signal may lead to Ca 2+ binding at the C1 site and, in turn, may be sufficient for partial activation of the channel [21] . On the other hand, ionic or metabolic conditions that weaken inhibitory coupling would result in increased Ca 2+ affinity at C3, and thus lead to greater channel activation in response to an equivalent Ca 2+ signal. The carboxyl–carboxylate bond between E133 and E259 would require at least partial protonation of these side chains; thus, with decreased [H + ] (that is, elevated pH), one would expect these side chains to become deprotonated and thus negatively charged. If both E133 and E259 were negatively charged, they would electrostatically repel one another, and the inhibitory coupling would be weakened. Ca 2+ activation of MthK is known to be greater with decreased [H + ]; thus, this mechanism could account for a component of the H + sensitivity of MthK gating, although other mechanisms may be involved [10] , [19] , [21] . Similar to MthK, the eukaryotic BK channel also contains RCK domains that are modulated by multiple, separate Ca 2+ -binding sites [13] , [32] , [33] . Functional analyses of the BK channel gating indicates that these separate binding sites can interact energetically [34] ; however, the structural basis of these interactions is not yet clear. As the BK channels are thought to be regulated by a number of potential physiological modulators, including H + , haem, carbon monoxide, nitric oxide and phosphorylation [35] , it will be important to apply structural analysis to better understand mechanisms underlying gating and modulation in these and other families of ion channels. Channel purification and reconstitution The full-length MthK channel, containing a C-terminal thrombin cleavage site followed by a 6xHis-tag, was expressed in Escherichia coli XL-1 Blue cells on induction with 0.4 mM IPTG (isopropyl β- D -1-thiogalactopyranoside) [10] . Bacteria were collected and resuspended in 20 mM Tris, 100 mM KCl, pH 7.6 (Buffer A), and lysed by sonication in the presence of phenylmethylsulphonyl fluoride and a protease inhibitor cocktail (Complete EDTA-free, Roche). The protein was solubilized by 2 h incubation in Buffer A with 50 mM decyl maltoside (DM), followed by centrifugation at 30,500 g for 45 min. The supernatant was loaded onto a Co 2+ -charged HiTrap metal affinity column (GE Healthcare), washed with 20 mM imidazole and 5 mM DM in Buffer A, and the channel protein was eluted using 400 mM imidazole and 5 mM DM in Buffer A. The 6xHis-tag was cleaved immediately after elution by incubating with 2.0 units of thrombin/3.0 mg eluted protein for 2 h at room temperature. Protein was concentrated using a centrifugal filtration unit (50 kDa molecular weight cut-off value) and further purified on a Superdex 200 gel filtration column, then concentrated again to 5 mg ml −1 . Channels were reconstituted into liposomes composed of E. coli lipids (Avanti) [36] , and the proteoliposomes were rapidly frozen in liquid N 2 and stored at −80 °C until use. Mutations were generated using the QuickChange Site-directed Mutagenesis Kit (Stratagene) and confirmed by DNA sequencing. Electrophysiology Recordings were obtained using planar lipid bilayers of POPE:POPG (3:1), in a horizontal bilayer chamber, at 22–24 °C. Solution in the cis (top) chamber contained 200 mM KCl and 10 mM HEPES, pH 7.0; solution in the trans (bottom) chamber contained 200 mM KCl, with either 10 mM HEPES (to buffer solutions to 7.7) or 10 mM 2-( N -morpholino)ethanesulfonic acid (MES) (to buffer solutions to pH 6.5), and CaCl 2 or CdCl 2 at the indicated concentrations. Recordings analysed for this work were obtained at −100 mV transmembrane voltage, although currents through each bilayer were observed at additional voltages to confirm the reversal potential and other MthK channel properties [37] . Within each bilayer, multiple solution changes were performed using a gravity-fed perfusion system, and to ensure completeness of solution changes the trans chamber was washed with a minimum of ten chamber volumes of solution before recording under a given set of conditions. Currents were amplified using a Dagan PC-ONE patch-clamp amplifier with low-pass filtering to give a final effective filtering of 1 kHz (dead time of 0.18 ms) and were sampled by computer at a rate of 10 kHz. Currents were analysed by measuring durations of channel openings and closings at each current level by 50% threshold analysis, using pClamp9. These measurements were used to quantify channel activity as NPo= , where i is the open level and P i is the per cent of time at that level. The mean channel open probability (Po) is then calculated by dividing N Po times N , which is the number of active channels in the bilayer, determined by recording under conditions where maximal channel opening is observed. Data are presented as mean±s.e.m. EC 50 values were estimated by fitting Po versus [Ca 2+ ] or Po versus [Cd 2+ ] data for individual bilayer patches using: Po=Po max /(1+([X 2+ ]/EC 50 ) n H), where Po max is the estimated maximum Po for the data set, [X 2+ ] is [Ca 2+ ] or [Cd 2+ ], EC 50 is the [Ca 2+ ] or [Cd 2+ ] yielding half-maximal activation and n H is the Hill coefficient. EC 50 values reported for each mutant are thus the means of EC 50 values determined from individual patches±s.e.m. Electrophysiological results are based on observations from a minimum of five different lipid bilayer patches for each recording condition and includes a total of 324 individual data sets from 67 different lipid bilayer patches. Crystallization WT and mutant MthK RCK domains, containing a C-terminal thrombin cleavage site followed by a 6xHis-tag, were expressed in E. coli BL-21(DE3) cells on induction with 0.4 mM IPTG [16] . Bacteria were collected and resuspended in 20 mM Tris, 250 mM NaCl, pH 7.6 (Buffer B), and lysed by sonication in the presence of phenylmethylsulphonyl fluoride and a protease inhibitor cocktail (Complete EDTA-free, Roche), followed by centrifugation at 30,500 g for 45 min. After adjusting the pH to 7.6, the supernatant was loaded onto a Co 2+ -charged HiTrap metal affinity column (GE Healthcare), washed with 20 mM imidazole in Buffer B and the channel protein was eluted using 400 mM imidazole in Buffer B. The 6xHis-tag was cleaved immediately after elution by incubating with 2.0 units of thrombin/3.0 mg eluted protein for 2 h at room temperature. The digested protein was then loaded onto a Superdex 200 gel filtration column and eluted with 20 mM Tris, 250 mM NaCl, pH 8.0. The eluted protein solution was concentrated to 6 mg ml −1 using a centrifugal concentrator (10 kDa molecular weight cut-off value) and the concentrated protein was aliquotted and stored in liquid N 2 until use. Crystals were formed in 2-μl hanging drops consisting of equal volumes of protein solution (6 mg ml −1 of purified MthK RCK domain, 250 mM NaCl, 20 mM Tris, pH 8.0) and crystallization buffer (6–12% polyethylene glycol 4,000, 1 M ammonium formate, 100 mM sodium acetate, pH 4.8, and 0.2–1 M calcium chloride, as indicated). Calcium chloride concentrations in the crystallization buffers were (in M): WT-C1, 0.2; E212Q, 0.2; D184N, 0.3; and WT-C1C2C3, 1.0. Crystals were mounted in nylon loops and rapidly frozen in liquid N 2 without additional cryoprotection, and then stored in liquid N 2 until the time of diffraction data collection. X-ray data collection and analysis Diffraction data were collected at beamline X6A (WT-C1) or X25 (WT-C1C2C3, D184N and E212Q) at the National Synchrotron Light Source, at 100 K under a nitrogen stream, at a wavelength of 1.1 Å. Data were processed and scaled using HKL2000 or iMosflm, and phasing was done by molecular replacement with Phaser using the unliganded MthK RCK domain structure (PDB accession number 2AEJ ) as the search model [38] , [39] . The final models for WT-C1 and WT-C1C2C3 each contained one RCK dimer (two peptide chains) per asymmetric unit, and final models for the D184N and E212Q mutants contained three RCK dimers (six peptide chains) per asymmetric unit. Examination of electron density maps and additional model building was performed using COOT, and models were refined by positional, isotropic B-factor and Translation/Libration/Screw refinement in Phenix [40] , [41] . To increase the observation:parameter ratio, torsion-angle non-crystallographic symmetry restraints were included in refinement for all but the WT-C1 structure. For the D184N and E212Q structures, which were refined using six NCS groups, bias in the assignment of the R free test sets was minimized by the use of thin resolution shells in test set selection, also performed using Phenix. Ramachandran plot analysis for each structure yielded (% in most favoured, allowed and disallowed regions): WT-C1C2C3 (98.2, 1.8, 0.0), WT-C1 (97.3, 2.7, 0.0), D184N (98.7, 1.3, 0.0) and E212Q (98.6, 1.4, 0.0). Omit maps were generated by deleting Ca 2+ ions and surrounding side chains, followed by two cycles of simulated annealing refinement, using Phenix. Figures were prepared using PyMOL. Accession codes: Coordinates and structure factors have been deposited in the RCSB protein databank under accession codes 4L73, 4L74, 4L75 and 4L76. How to cite this article: Smith, F. J. et al . Structural basis of allosteric interactions among Ca 2+ -binding sites in a K + -channel RCK domain. Nat. Commun. 4:2621 doi: 10.1038/ncomms3621 (2013).